Biocompatible click chemistry enabled compartment-specific pH measurement insideE. coli Bioorthogonal reactions, especially the Cu(I)-catalysed azide–alkyne cycloaddition, have revolutionized our ability to label and manipulate biomolecules under living conditions. The cytotoxicity of Cu(I) ions, however, has hindered the application of this reaction in the internal space of living cells. By systematically surveying a panel of Cu(I)-stabilizing ligands in promoting protein labelling within the cytoplasm of Escherichia coli , we identify a highly efficient and biocompatible catalyst for intracellular modification of proteins by azide–alkyne cycloaddition. This reaction permits us to conjugate an environment-sensitive fluorophore site specifically onto HdeA, an acid-stress chaperone that adopts pH-dependent conformational changes, in both the periplasm and cytoplasm of E. coli . The resulting protein–fluorophore hybrid pH indicators enable compartment-specific pH measurement to determine the pH gradient across the E. coli cytoplasmic membrane. This construct also allows the measurement of E. coli transmembrane potential, and the determination of the proton motive force across its inner membrane under normal and acid-stress conditions. Both eukaryotic and prokaryotic cells are compartmentalized. Inside eukaryotic cells, metabolic processes and signalling events are frequently carried out in the cytosol or specialized organelles (for example, mitochondria, ER and Golgi), with well-defined pH and oxidative status. Although to a lesser extent, the intracellular space of Gram-negative bacteria is also compartmentalized as cytoplasmic and periplasmic spaces, with the latter separated from the environment and the cytoplasm by a highly porous outer membrane and a tighter inner membrane (or cytoplasmic membrane), respectively. This arrangement produces a distinct environment within these bacterial compartments under normal and stress conditions. For example, enteric pathogens such as Escherichia coli and Shigella spp. have to pass through the highly acidic human stomach (pH<3) before reaching their primary infection site in the small intestine [1] , [2] . To survive this acidic environment, E. coli cells have evolved multiple acid-resistance systems to elevate their internal pH [3] , including generating a pH gradient across the cytoplasmic membrane. The pH gradient (ΔpH=pH cytoplasm −pH periplasm ) is a key component of the proton motive force ( PMF ), which, in conjunction with the membrane potential (Δ Ψ ), determines the electrochemical gradient, namely PMF , across E. coli cytoplasmic membrane [4] . Many biological processes are energetically linked to the free energy produced by PMF , including ATP synthesis, the transport of nutrients across the cytoplasmic membrane, as well as the rotation of bacterial flagella [5] , [6] . There are currently no suitable indicators for measuring pH gradient under acid-stress, since small molecule fluorophores lack targeting specificity while pH-sensitive fluorescent proteins denature below pH5 (refs 7 , 8 ). Therefore, the ability to directly target pH indicators into different E. coli compartments is highly desired. Coupling the genetic code expansion strategy with bioorthogonal chemistry provides a powerful tool for highly specific protein labelling in vitro and in living cells. For example, an unnatural amino acid bearing a bioorthogonal handle can be genetically incorporated into a given protein that is expressed in a specific location, allowing the subsequent bioorthognal labelling with a small molecule fluorophore. However, this strategy has largely focused on in situ labelling of biomolecules topologically located on the surface of mammalian or bacterial cells [9] , [10] , or within the bacterial periplasm [11] , [12] . Protected by single or double plasma membranes, molecules located in the highly reduced and fragile cytoplasm represent attractive yet challenging targets for bioorthogonal labelling. Currently, the state-of-the-art bioorthogonal click reactions include the Cu(I)-catalysed azide–alkyne cycloaddition (CuAAC) and the strain-promoted azide–alkyne cycloaddition (SPAAC), among a few others [13] , [14] , [15] . In their pioneering work on SPAAC, Tirrell, Bertozzi and co-workers found that, when cyclooctyne-based fluorescent probes was used to label newly synthesized proteins in live mammalian cells [16] , a high fluorescence background was observed, which was later attributed to the nonspecific reactivity of the DIFO probe toward free thiols or cysteine-containing proteins [17] , [18] . Notably, several studies have shown that CuAAC exhibited 10−100 times faster kinetics than SPAAC in aqueous solutions, and that the terminal alkyne is an excellent bioorthogonal handle [19] , [20] . These attributes make CuAAC an attractive candidate for in vivo labelling. However, copper is known to be toxic to both eukaryotic and prokaryotic cells. For example, copper destroys many biomolecules by oxidative damage, and thus, E. coli compartmentalizes its copper-dependent enzymes in the periplasm as well as the outer aspect of the cytoplasmic membrane, leaving an extremely low level of copper in the reduced cytoplasm [21] . Furthermore, several recent studies showed that the highly thiophilic Cu(I) ions can directly impair Fe-S cluster-containing enzymes located exclusively within the bacterial cytoplasm, which has been suggested as a major lethal effect of copper inside microorganisms [22] , [23] . Interestingly, these same studies indicated that sequestration of copper ions by chelators such as bathocuproine sulphonate or copper-binding proteins can restrict the tendency of copper to damage intracellular Fe-S clusters, and thus enhance bacterial tolerance to copper. These observations, together with our recent success in the discovery of accelerating ligands that render CuAAC biocompatible for labelling cell-surface glycans in living organisms [24] , [25] , prompted us to explore the feasibility of utilizing the ligand-assisted CuAAC to label cytoplasmic proteins within living bacterial cells. Herein, we report that tris(triazolylmethyl)amine-coordinated Cu(I) catalysts, BTTP–Cu(I) and BTTAA–Cu(I), permit the in situ labelling of azide-incorporated proteins in the cytoplasm of E. coli without apparent toxicity. Employing this biocompatible ligation chemistry, we specifically targeted a protein–fluorophore hybrid pH indicator into the E. coli cytoplasm for internal pH measurement. By employing both the cytoplasm- and periplasm-residing pH indicators, we determine the pH values in these two compartments under highly acidic conditions. The calculated pH gradient (ΔpH) across E. coli cytoplasmic membrane, in conjunction with the measured transmembrane potential (Δ Ψ ) using a Δ Ψ -sensitive dye, enable us to obtain the PMF value across E. coli cytoplasmic membrane under acid-stress conditions. Ligand-assisted CuAAC for protein labelling in bacterial cytoplasm As the first step to evaluate CuAAC as a biocompatible tool to label cytosolic proteins in E. coli , we chose a cytosolically expressed green fluorescent protein (GFP) bearing a single azide handle as the model system. A panel of Cu(I)-stabilizing ligands developed by us and others were surveyed to assess their efficiency in promoting the CuAAC-mediated protein labelling ( Fig. 1a ). TBTA, the canonical ligand developed by Sharpless and co-workers, is the most commonly used ligand for bioorthogonal conjugation [26] . However, TBTA has poor solubility in aqueous buffer, resulting in incomplete ligation when azide and alkyne are at micromolar concentrations [27] . BTTAA and BTTPS are two water soluble TBTA analogues. Both ligands dramatically accelerate CuAAC and render it biocompatible for labelling cell-surface glycans and proteins in live zebrafish embryos [24] , [25] . As an unsulphated version of BTTPS, BTTP exhibited a similar efficiency as BTTPS in promoting CuAAC-mediated protein in vitro labelling [25] . Finally, we also examined bathophenanthroline disulphonate (BPS), a well-known negatively charged Cu(I)-chelator, as well as L -histidine, a recently reported effective ligand for accelerating CuAAC to label mammalian cell-surface glycans [28] , [29] . 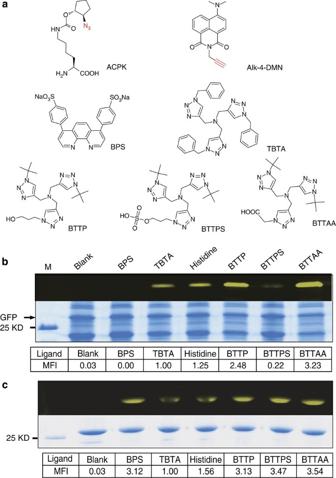Figure 1: Comparison of the labelling efficiencyin vitroand within theE. colicytoplasm. (a) Structures of the Pyl analogue ACPK, the alkyne-tethered fluorophore alk-4-DMN as well as Cu(I)-stabilizing ligands for CuAAC reaction used in this study. ACPK,Nε-((1R,2R)-2-azidocyclopentyloxy)carbonyl)-L-lysine; BPS, bathophenanthroline disulphonate disodium salt; BTTAA, 2-[4-{(bis[(1- tert-butyl-1H-1,2,3-triazol-4-yl)methyl]amino)methyl}-1H-1,2,3-triazol-1-yl]-acetic acid; BTTP, 3-[4-({bis[(1-tert-butyl-1H-1,2,3-triazol-4-yl)methyl]amino}methyl)- 1H-1,2,3-triazol-1-yl]propanol; BTTPS, 3-[4-({bis[(1-tert-butyl-1H-1,2,3-triazol-4- yl)methyl]amino}methyl)-1H-1,2,3-triazol-1-yl]propyl hydrogen sulphate; 4-DMN: 4-N,N-dimethyl amino-1,8-naphthalimide; TBTA, tris-((1-benzyl-1H-1,2,3-triazol-4-yl)methyl)amine. (b,c) Efficiency ofin vivo(b) andin vitro(c) protein labelling mediated by ligand-assisted CuAAC. The reaction products between GFP-N149-ACPK and alk-4-DMN were analysed by SDS–PAGE and visualized under ultraviolet illumination (top) before being stained by Coomassie blue (bottom). Blank, without Cu(I) catalyst; M, protein marker; MFI, mean fluorescence intensity. Figure 1: Comparison of the labelling efficiency in vitro and within the E. coli cytoplasm. ( a ) Structures of the Pyl analogue ACPK, the alkyne-tethered fluorophore alk-4-DMN as well as Cu(I)-stabilizing ligands for CuAAC reaction used in this study. ACPK, N ε -((1R,2R)-2-azidocyclopentyloxy)carbonyl)- L -lysine; BPS, bathophenanthroline disulphonate disodium salt; BTTAA, 2-[4-{(bis[(1- tert-butyl-1H-1,2,3-triazol-4-yl)methyl]amino)methyl}-1H-1,2,3-triazol-1-yl]-acetic acid; BTTP, 3-[4-({bis[(1-tert-butyl-1H-1,2,3-triazol-4-yl)methyl]amino}methyl)- 1H-1,2,3-triazol-1-yl]propanol; BTTPS, 3-[4-({bis[(1-tert-butyl-1H-1,2,3-triazol-4- yl)methyl]amino}methyl)-1H-1,2,3-triazol-1-yl]propyl hydrogen sulphate; 4-DMN: 4- N,N -dimethyl amino-1,8-naphthalimide; TBTA, tris-((1-benzyl-1H-1,2,3-triazol-4-yl)methyl)amine. ( b , c ) Efficiency of in vivo ( b ) and in vitro ( c ) protein labelling mediated by ligand-assisted CuAAC. The reaction products between GFP-N149-ACPK and alk-4-DMN were analysed by SDS–PAGE and visualized under ultraviolet illumination (top) before being stained by Coomassie blue (bottom). Blank, without Cu(I) catalyst; M, protein marker; MFI, mean fluorescence intensity. Full size image The azide-bearing GFP (GFP-N149-ACPK), constructed by site-specific incorporation of a pyrrolysine (Pyl) analogue bearing an azide residue, ACPK ( Fig. 1a ), into residue 149 via our previously evolved pyrrolysyl-tRNA synthetase-tRNA pair, was expressed in E. coli . We performed the ligation chemistry by incubating live E. coli cells harbouring GFP-N149-ACPK with alk-4-DMN in the presence of the aforementioned panel of copper ligands at room temperature for 1 h ( Fig. 1b , Supplementary Figs 1–4 ). The lysates of cells were resolved by SDS–polyacrylamide gel electrophoresis (SDS–PAGE) and analysed by in-gel fluorescence. As shown in Fig. 1b , BTTP–Cu(I) and BTTAA–Cu(I) exhibited the highest reactivity in catalyzing this in vivo protein labelling process; the yield of BTTP–Cu(I)-mediated reaction was at least sevenfold higher than that achieved by using the uncoordinated Cu(I) ( Supplementary Fig. 5 ). Approximately two- to threefold lower activity was observed in the TBTA–Cu(I) and L -histidine-Cu(I) catalysed reactions. By contrast, BTTPS–Cu(I) yielded an extremely low amount of fluorescently labelled proteins and no detectable fluorescent product was obtained in the BPS–Cu(I) mediated reaction. These results were in direct contrast to the data obtained from the in vitro labelling experiments ( Fig. 1c ), in which equal quantity of GFP-N149-ACPK was reacted with alk-4-DMN in the presence of the same set of Cu(I) complexes. In the in vitro labelling experiments, BPS–Cu(I) and BTTPS–Cu(I) produced similar levels of ligation products compared with that of BTTP–Cu(I) and BTTAA–Cu(I), whereas TBTA and L -histidine exhibited two- to threefold lower labelling efficiency than the remaining four ligands. In addition, the GFP protein still retained about 95% of its fluorescence intensity after the treatment with BTTP–Cu(I) and BTTAA–Cu(I), indicating that these Cu(I) complexes had little influence on its structural integrity ( Supplementary Fig. 6 ). The difference between the efficiency of Cu(I) catalyst-assisted click labelling of GFP-N149-ACPK in vitro and within living E. coli cells suggests that even though the same concentrations of ligand–Cu(I) complexes were used, their working concentrations in bacterial cytoplasm might be significantly varied. To test this hypothesis, we employed ICP–AES (inductively coupled plasma–atomic emission spectrometry) to measure the copper concentration within E. coli cytoplasm upon treatment with these Cu(I) complexes ( Supplementary Methods and Fig. 2a ). We isolated the cytoplasmic fraction of bacteria using an osmotic shock method to avoid contamination by copper from the periplasm ( Supplementary Fig. 7 ). ICP–AES analysis on these cytoplasmic samples and whole-cell samples showed that the bacterial cells exhibited apparent preference towards certain copper sources. More copper was present in E. coli cytoplasm when treated with free Cu(I) ions than with an equal amount of ligand–Cu(I) complexes. As expected, BPS–Cu(I) and BTTPS–Cu(I) were taken up by the cells less effectively compared with other Cu(I) complexes because the negatively charged sulphate group on BPS and BTTPS significantly decreased their membrane permeability. This observation, combined with the aforementioned in vivo labelling results, suggest that the low labelling efficiency observed in the BPS–Cu(I) and BTTPS–Cu(I) catalysed reactions was likely due to the low level of these Cu(I) complexes delivered into the cytoplasm. Importantly, although the other four Cu(I) complexes resulted in equimolar Cu(I) concentration within the cytoplasm, their ability to promote the CuAAC labelling reaction varied significantly, with BTTP and BTTAA possessing two- to threefold higher efficiency than the other two ligands. Taken together, our results indicated that, at equal concentration of Cu(I), BTTP and BTTAA served as the best ligands for accelerating CuAAC reaction in the bacterial cytoplasm. 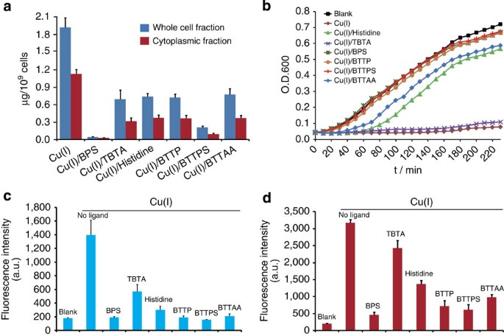Figure 2: Toxicity of Cu(I) complexes insideE. colicells. (a) Metal uptake of Cu(I)–ligand complexes in theE. colicytoplasm. Both the whole-cell fraction (blue columns) and the cytoplasmic fraction (red columns) were subjected to copper content measurement by ICP–AES. Error bars, s.d. from three independent experiments. (b)E. coligrowth curves after being treated with different Cu(I)–ligands. Blank,E. colicells without Cu(I) treatment. The data are representative of three independent experiments. (c) Detection of intracellular generation of ROS fromE. colicells using DCFH-DA as the reporter. Blank,E. colicells without Cu(I) treatment. Error bars, s.d. from three independent experiments. (d) Fluorescence of PI-stainedE. colicells after being treated with Cu(I) ligands for 1 h. Blank,E. colicells without Cu(I) treatment. Error bars, s.d. from three independent experiments. Figure 2: Toxicity of Cu(I) complexes inside E. coli cells. ( a ) Metal uptake of Cu(I)–ligand complexes in the E. coli cytoplasm. Both the whole-cell fraction (blue columns) and the cytoplasmic fraction (red columns) were subjected to copper content measurement by ICP–AES. Error bars, s.d. from three independent experiments. ( b ) E. coli growth curves after being treated with different Cu(I)–ligands. Blank, E. coli cells without Cu(I) treatment. The data are representative of three independent experiments. ( c ) Detection of intracellular generation of ROS from E. coli cells using DCFH-DA as the reporter. Blank, E. coli cells without Cu(I) treatment. Error bars, s.d. from three independent experiments. ( d ) Fluorescence of PI-stained E. coli cells after being treated with Cu(I) ligands for 1 h. Blank, E. coli cells without Cu(I) treatment. Error bars, s.d. from three independent experiments. Full size image Toxicity study of Cu(I) complexes to E. coli Next, we investigated the toxicity of these Cu(I) complexes to E. coli cells by using a proliferation assay. As shown in Fig. 2b , similar to the uncoordinated Cu (I) ions, the TBTA–Cu(I) complex dramatically inhibited bacterial proliferation. By contrast, all the other ligands attenuated copper toxicity to a certain extent. In particular, BTTPS–Cu(I) and BTTP–Cu(I) imparted negligible influences on bacterial growth. To evaluate the potential harmful effects from these Cu(I) complexes after a longer incubation time, a plate sensitivity assay was also performed on bacterial cells treated with the same panel of Cu(I) copper complexes overnight, which yielded similar results ( Supplementary Fig. 8 ). The low toxicity of BTTPS might be due to its low membrane permeability whereas BTTP and BTTAA might effectively block the damaging effects of Cu(I) to essential intracellular proteins such as Fe-S cluster-containing enzymes. To determine if this ligand coordination attenuates the damage of Fe-S cluster-containing enzymes by Cu(I) ions, we adopted a cell-growth assay using E. coli GR17 strain that lacks copper homeostatic systems ( copA::kan Δ c ueO Δ cusCFBA::cm ) developed by Imlay and co-workers [22] ( Supplementary Fig. 9 ). Treatment with 10 μM of uncoordinated Cu(I) was sufficient to inhibit the growth of GR17 cells, whereas inclusion of the ligands BTTP or BTTAA restored cell growth almost to the same level as the addition of branched-chain amino acids. These results further confirmed that BTTP and BTTAA could largely sequester Cu(I) induced damage of Fe-S cluster-containing enzymes such as isopropylmalate dehydratase involved in the biosynthesis of branched-chain amino acids. The mechanism of copper-associated cytotoxicity remains elusive. A long-standing hypothesis is that Cu(II)/Cu(I) ion redox chemistry mediates the production of reactive oxygen species (ROS) [30] such as the highly deleterious hydroxyl radicals, which may cause damages to the cell membrane and Fe-S cluster-containing enzymes [22] . We used a commercial fluorogenic assay to assess if ligand coordination attenuates the production of hydroxyl radicals generated by Cu(I) [31] ( Supplementary Fig. 10 ). All ligands examined reduced ROS production to a certain degree, with BTTPS and BTTP exhibiting the highest efficiency. Furthermore, we directly analysed the Cu(I)-mediated ROS production inside E. coli cells by using a hydroxyl radical-sensitive fluorescent probe 2′,7′-dichlorofluorescein (DCF) as the reporter [32] ( Fig. 2c ). Whereas the ligand-free Cu(I) ions generated a sevenfold increase in intracellular ROS compared with untreated cells, TBTA–Cu(I) showed only a threefold fluorescence increase and all other Cu(I) complexes exhibited a <1.5-fold fluorescence change. Effect of Cu(I) complexes on membrane integrity Maintaining cell membrane integrity is critical for bacterial physiology. Accordingly, it is important to develop an accurate measurement of pH gradient and PMF values across the E. coli membrane. To ascertain the integrity of E. coli membrane upon treatment with Cu(I) complexes, we incubated the bacteria with each of the six Cu(I) catalysts ([Cu]=100 μM, [ligand]=200 μM) for 1 h at room temperature, followed by propidium iodide (PI) staining [33] ( Fig. 2d ). Severe membrane damage was observed when cells were treated with either uncoordinated Cu(I) or Cu(I)–TBTA complex. The remaining Cu(I) ligands all effectively attenuated copper’s damage to the membrane. Similar results were obtained when trypan blue [34] , another commonly used fluorescent dye to assess cell viability, was used ( Supplementary Methods and Supplementary Fig. 11 ). The propensity for ROS production by these Cu(I) catalysts correlates well with their membrane damaging effects. Our in vitro and in vivo experiments demonstrate that uncoordinated Cu(I) was highly active in generating detrimental hydroxyl radicals, whereas ligand-coordinated Cu(I) complexes produced much lower levels of oxidative species and thus less toxic. This is likely because the ligand may actively adjust the redox potential of Cu(I) ions through coordination. In theory, the higher the redox potential, the lower the propensity of Cu(I) complexes in generating ROS [35] . To examine whether our aforementioned findings are consistent with this principle, we measured the redox potentials of BTTPS–Cu(I), BTTP–Cu(I) and BTTAA–Cu(I) complexes and compared our results with the well-documented redox potential of the uncoordinated Cu(I). As shown in Table 1 and Supplementary Fig. 12 , the measured redox potentials of BTTPS–Cu(I) and BTTP–Cu(I) were approximately 40 mV higher than that of BTTAA–Cu(I), which, in turn, was 90 mV higher than the value of the uncoordinated Cu(I). Table 1 Electrochemical data of Cu(I) complex in H 2 O. Full size table Taken together, our experiments confirmed that the ligand-free Cu(I) and TBTA-complexed Cu(I) were highly toxic to E. coli cells and that BPS- and BTTPS-complexed Cu(I) exhibited low toxicity, likely due to the negatively charged sulphate group that blocks their cellular entry. However, this same feature also rendered these two catalysts unsuitable for intracellular applications. Consistent with the previous study in mammalian cells, L -histidine was found to attenuate copper-associated toxicity in E. coli . However, its ability to accelerate CuAAC is considerably lower than the water soluble tris(triazolylmethyl)amine-based ligands. In addition, there are concerns that L -histidine may serve as a solubilizing agent for Cu(I) to facilitate damaging of essential Fe-S clusters of dehydratases [22] . By increasing the redox potential of the coordinated Cu(I), BTTP and BTTAA significantly reduced the production of ROS as well as the damaging effects to cell membrane. These ligands also efficiently blocked the damage of Cu(I) to intracellular Fe-S cluster containing enzymes. Together, excellent biocompatibility inside living bacterial cells can be achieved with BTTP and BTTAA. In particular, when compared with the BTTAA–Cu(I) complex that we have previously used [12] , we found that BTTP–Cu(I) exhibited a further lowered ROS production, cellular damage and toxicity in assisting CuAAC-mediated protein labelling inside living E. coli cells. This sets up the stage for applying BTTP–Cu(I) complex for protein labelling within internal spaces of live bacterial cells. Retargeting a periplasmic pH indicator into the cytosol To demonstrate the applications of BTTP-assisted CuAAC for intracellular protein labelling beyond GFP, we applied this biocompatible ligation chemistry to target a previously developed, periplasm-located protein-small molecule pH indicator into the E. coli cytoplasm. Enteric pathogens such as E. coli have to pass through the highly acidic human stomach (pH<3) before reaching their primary infection site in the small intestine. Due to the highly porous nature of the bacterial outer membrane, the periplasmic space is believed to rapidly equilibrate with the acidic extracellular environment [7] , [36] . In contrast, the cytoplasm is buffered at a much higher pH level, thereby generating an intracellular pH gradient that is crucial for the survival of enteric bacteria during acid-stress. Compartment-specific pH indicators derived from the same fluorphore or fluorescent protein is advantageous for quantitative comparison of pH values within different intracellular spaces, mainly due to their unified chemical nature and pH response features. However, in contrast to many organelle-specific derivatives of a pH indicator that is applicable to different mammalian compartments, it remains a challenge to directly target a unified indicator into different bacterial spaces for pH measurement. The pH-responsive fluorescent proteins are largely restricted to the E. coli periplasm due to the difficulty for cytoplasmic-membrane trafficking, as well as the low efficiency in folding of these fluorescent proteins in the oxidized periplasm. Furthermore, most of these pH-sensitive proteins will be denatured when the pH drops to <5, rendering them incapable of measuring highly acidic environment that resembles those met in the human stomach. In addition, most small molecule fluorophores lack targeting specificity to discriminate between the bacterial periplasm and cytoplasm. The membrane permeable fluorophores may occupy both spaces, whereas bulky or negatively charged fluorophores are inaccessible to the cytoplasm due to the tight cytoplasmic inner-membrane space. Therefore, the lack of a unified indicator suitable for pH measurement in different internal bacterial spaces renders the internal pH gradient of E. coli cells rather elusive, particularly under acid-stress conditions. We recently developed a periplasm-localizing, protein–fluorophore hybrid pH indicator by applying BTTAA-assisted CuAAC between an alkyne-bearing solvatochromic fluorophore (alk-4-DMN) and a periplasm-expressing acid chaperone HdeA, with ACPK incorporated as residue 58 within its pH-responsive region [12] (peri-HdeA-58-ACPK; Fig. 3a ). The resulting periplasm-residing pH indicator, termed peri-pHin, was able to operate under a wide pH range, permitting us to specifically measure the acidity of the E. coli periplasm when the extracellular pH varied from neutral to pH 2. Because removal of the amino (N)-terminal signalling peptide can redirect HdeA from the periplasm to the cytoplasm [12] and our BTTP–Cu(I) complex is highly compatible with the cytoplasm, we employed BTTP-assisted CuAAC to label the cytosolic version of ACPK-bearing HdeA protein (cyto-HdeA-58-ACPK) with alk-4-DMN. The proper localization of the resulting cytosolic pH indicator, termed cyto-pHin, was verified by immunoblotting analysis against the cytosolic as opposed to the periplasmic fraction of E. coli using an anti-HdeA antibody ( Fig. 3b ; Supplementary Fig. 13 ). Furthermore, the BTTP-assisted click-labelling efficiency and the specificity for producing both peri-pHin and cyto-pHin were confirmed by fluorometric SDS–PAGE analysis ( Fig. 3c ). In vitro fluorescence measurement showed that peri-pHin and cyto-pHin proteins have nearly the same pH response pattern ( Supplementary Fig. 14 ). Notably, by quantitatively comparing the protein expression levels and the corresponding fluorescence intensity from the two gel bands, the in vivo click-labelling efficiency of cyto-pHin was determined to be 0.94 as that of peri-pHin ( Supplementary Fig. 15 ). In addition, by quantitative comparison of the fluorescence intensity between peri-HdeA58-ACPK (or cyto-HdeA58-ACPK) proteins labelled by alk-4-DMN in E. coli cells and the in vitro quantitatively labelled HdeA58-DMN, we have calculated the in vivo labelling yield as 73 and 69% for peri-HdeA58-ACPK and cyto-HdeA58-ACPK, respectively ( Supplementary Fig. 16 ). 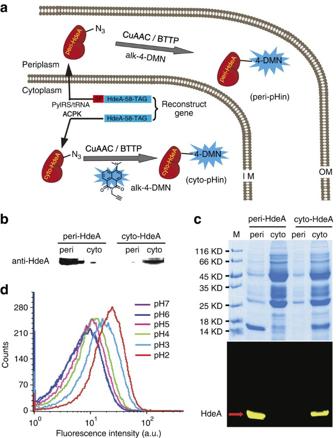Figure 3: Directing a genetically encoded click-labelled pH indicator to differentE. coliinternal spaces. (a) An acid chaperone protein HdeA with or without a periplasm-targeting signal peptide (SP) were expressed carrying a site-specifically incorporated azide-bearing unnatural amino acid, ACPK, as residue 58. The resulting proteins were then conjugated with alk-4-DMN via ligand-assisted CuAAC reaction to afford specific pH indicators inE. colicytoplasm (cyto-pHin) and periplasm (peri-pHin), respectively. IM, inner membrane (cytoplasmic membrane), OM, outer membrane, SP, signal peptide sequence. CuAAC: copper catalysed azide–alkyne cycloaddition. (b) Immunoblotting analysis showing the localization of peri-HdeA and cyto-HdeA. (c) Generation of compartment-specific pH indicators, peri-pHin and cyto-pHin, as analysed by SDS–PAGE. M, protein marker. (d) Flow cytometry results ofE. colicells harbouring cyto-pHin as a function of pH (7.0–2.0). Figure 3: Directing a genetically encoded click-labelled pH indicator to different E. coli internal spaces. ( a ) An acid chaperone protein HdeA with or without a periplasm-targeting signal peptide (SP) were expressed carrying a site-specifically incorporated azide-bearing unnatural amino acid, ACPK, as residue 58. The resulting proteins were then conjugated with alk-4-DMN via ligand-assisted CuAAC reaction to afford specific pH indicators in E. coli cytoplasm (cyto-pHin) and periplasm (peri-pHin), respectively. IM, inner membrane (cytoplasmic membrane), OM, outer membrane, SP, signal peptide sequence. CuAAC: copper catalysed azide–alkyne cycloaddition. ( b ) Immunoblotting analysis showing the localization of peri-HdeA and cyto-HdeA. ( c ) Generation of compartment-specific pH indicators, peri-pHin and cyto-pHin, as analysed by SDS–PAGE. M, protein marker. ( d ) Flow cytometry results of E. coli cells harbouring cyto-pHin as a function of pH (7.0–2.0). Full size image We next applied flow cytometry to measure the fluorescence of E. coli cells harbouring cyto-pHin under a wide range of extracellular acidity. The extracellular pH values were reduced step-wise from pH 7 to pH 2 followed by flow cytometric analysis at each pH value ( Fig. 3d ). A gradual increase in fluorescence signal was observed, and we plotted this fluorescence change against each pH unit. A total of threefold fluorescence enhancement in cyto-pHin signal was observed, which was smaller than that of peri-pHin (>fivefold), indicating that the cytosolic pH varied to a lesser extent than the periplasmic pH. Measuring pH gradient across the cytoplasmic membrane By employing our two compartment-specific pH indicators, peri-pHin and cyto-pHin, we next measured the pH gradient across E. coli cytoplasmic membrane under acid-stress conditions. Flow cytometric analysis was first performed on the peri-pHin-expressing cells under various external pH conditions with and without 20 mM benzoate, a membrane permeable weak acid that transports protons across the bacterial membranes to lower the internal pH [37] . Consistent with previous reports, our results revealed that the E. coli periplasmic pH showed negligible change in response to benzoate treatment when the extracellular pH was >5 (ref. 7 ). However, when the external pH dropped to <5, peri-pHin detected a small but noticeable change in fluorescence after the benzoate treatment; the presence of benzoate led to a further increase in fluorescence of peri-pHin ( Fig. 4a ). As a negative control, E. coli cells bearing the pH-insensitive variant peri-HdeA-72-DMN were subjected to flow cytometric analysis under different pH conditions, but exhibited essentially no fluorescence changes throughout all pH conditions in the presence and absence of 20 mM benzoate ( Supplementary Fig. 17 ). This led us to believe that the periplasmic space of E. coli might also be slightly buffered by basic amino acids and polyamines that are exported from the E. coli cytoplasm, particularly when surrounded by highly acidic environment such as gastric acid. 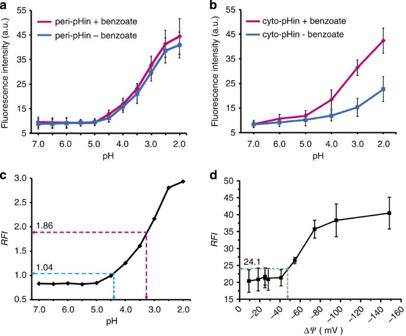Figure 4: Measuring the pH values inE. coliperiplasm and cytoplasm under acid stress. (a) The pH-dependent fluorescence response curves of peri-pHin in the presence and absence of 20 mM sodium benzoate. Error bars, s.d. from three independent experiments. (b) The pH-dependent fluorescence response curves of cyto-pHin in the presence and absence of 20 mM sodium benzoate. Error bars, s.d. from three independent experiments. (c) Calibration curve of extracellular pH as a function of relative fluorescence intensity (RFI). TheRFIwas generated as the ratio of the fluorescence intensity between peri-pHin and peri-HdeA-72-DMN (with benzoate) at each pH point. (d) Calibration curve of membrane potential (ΔΨ) as a function of relative fluorescence intensity (RFI) at pH 3. TheRFIwas generated as the ratio of the fluorescence intensity between the red and green channels. Figure 4: Measuring the pH values in E. coli periplasm and cytoplasm under acid stress. ( a ) The pH-dependent fluorescence response curves of peri-pHin in the presence and absence of 20 mM sodium benzoate. Error bars, s.d. from three independent experiments. ( b ) The pH-dependent fluorescence response curves of cyto-pHin in the presence and absence of 20 mM sodium benzoate. Error bars, s.d. from three independent experiments. ( c ) Calibration curve of extracellular pH as a function of relative fluorescence intensity ( RFI ). The RFI was generated as the ratio of the fluorescence intensity between peri-pHin and peri-HdeA-72-DMN (with benzoate) at each pH point. ( d ) Calibration curve of membrane potential (Δ Ψ ) as a function of relative fluorescence intensity ( RFI ) at pH 3. The RFI was generated as the ratio of the fluorescence intensity between the red and green channels. Full size image Next, we utilized E. coli cells harbouring cyto-pHin to monitor the cytoplasmic pH change in response to an increasing extracellular acidity from pH 7 to pH 2 with and without 20 mM benzoate ( Fig. 4b ). In contrast to the pH measurement in the periplasm, our analysis showed that the addition of benzoate enhanced the fluorescence under all pH conditions, consistent with the fact that the E. coli cytoplasm maintains a much higher buffering capacity than its periplasm. In particular, the bacterial fluorescence in the presence of benzoate increased significantly when the extracellular acidity was decreased to below pH 5, which indicated a stronger cytosolic buffering capacity upon the acidification of the extracellular environment. We also expressed the pH-insensitive HdeA control variant (HdeA-72-DMN) in the cytoplasm (cyto-HdeA-72-DMN), but observed no noticeable fluorescence differences under all pH conditions we tested with and without benzoate ( Supplementary Fig. 17 ). For quantitative measurement, we generated a calibration curve of the extracellular pH as a function of relative fluorescence intensity ( RFI , Fig. 4c ); the curve was further validated by a series of standard pH solutions ( Supplementary Fig. 18 ). Based on these pH-dependent flow cytometric investigations as well as the RFI derived from peri-pHin and cyto-pHin at a given pH buffer, we determined that the periplasmic pH was about 0.3 pH unit higher than the extracellular space when the environmental acidity was at pH 3.0. Under the same condition, E. coli cytosolic pH was calculated to be 4.4 ( Fig. 4c,d ), which is significantly higher than the environment or the cytoplasm after benzoate treatment ( Supplementary Fig. 19 ). Thus the pH gradient across the E. coli cytoplasmic membrane was about +1.1 pH unit when the extracellular pH was at 3. To further verify the reliability of our pH indicators, we incubated E. coli cells harbouring the cyto-peri-pH indicator in acidic M9 minimal medium (pH 3) or in an acidic buffer containing pepsin, a digestive enzyme that is present in the gastric acid environment of the human stomach. The subsequent flow cytometric analysis and calculation showed cytosolic pH values of 4.5 and 4.4, respectively, which were similar to the pH value when E. coli was surrounded by pH 3 citrate buffer ( Supplementary Fig. 20 ). Taken together, these results indicated that the digestive enzymes and inorganic salts present in biological systems were not interfering with our pH indicators. PMF determination across the E. coli cytoplasmic membrane To obtain the PMF value across the E. coli cytoplasmic membrane, we next employed a ratiometric fluorescent probe for measurement of Δ Ψ in E. coli cells by using flow cytometry. DiOC 2 (3) is a lipophilic cyanine dye with a delocalized positive charge [38] , [39] . Upon excitation by a 488-nm laser, the fluorescence of the stained cells could be detected in both the green channel (530 nm) and red channel (>600 nm). The green fluorescence is dependent on cell size but independent of Δ Ψ ; while the red fluorescence, due to the formation of dye aggregates, is dependent on both cell size and Δ Ψ . The ratio of red to green fluorescence would thus provide an accurate measurement of membrane potential. To calibrate the values of the calculated fluorescence ratio to that of Δ Ψ , the DiOC 2 (3)-stained E. coli cells were treated with potassium-specific ionophore, valinomycin, in the presence of different concentrations of external potassium ions [38] , [40] . Membrane potential was calculated from K + distribution across the cytoplasmic membrane by means of the Nernst equation [41] . In this way, we generated the calibration curves of relative fluorescence intensity ( RFI , red fluorescence intensity/green fluorescence intensity) as a function of Δ Ψ at the extracellular pH 7 and pH 3 ( Supplementary Fig. 21 and Fig. 4d ). At pH 7, the RFI was a valid indicator of Δ Ψ in the range of −105 mV through −145 mV; whereas the RFI −Δ Ψ was accurate between −40 and −80 mV at pH 3. On the basis of the flow cytometric analysis of DiOC 2 (3)-stained E. coli cells both under neutral and acidic extracellular conditions, we determined that the membrane potential of E. coli was −124 mV when the environment was at pH 7, which is consistent with previous reports [41] . In contrast, Δ Ψ decreased to −47 mV when the extracellular acidity dropped to pH 3, probably due to the acid-stress-induced depolarization of E. coli cell membrane [42] . Finally, we calculated the PMF across E. coli cytoplasmic membrane under both neutral and acidic conditions. According to the equation PMF (mV)=Δ Ψ −59 × ΔpH in Table 2 , the PMF was calculated as −159 mV at pH 7 ( Supplementary Fig. 21 ). In contrast, when the extracellular acidity dropped to pH 3, the PMF value was calculated to be −112 mV, which is smaller in magnitude than that at pH 7. Therefore, when the external pH decreased from neutral to pH 3, the Δ Ψ across the E. coli cytoplasmic membrane dramatically decreased from −124 to −47 mV, whereas the ΔpH values increased about 1.1 pH unit. Together, the PMF value across the E. coli cytoplasmic membrane underwent a relatively small decrease from −159 to −112 mV, which is still highly negative. Table 2 PMF of Escherichia coli cells under extreme acidic conditions (pH 3). Full size table Using a newly developed Cu(I) ligand in assisting the CuAAC reaction, we have achieved highly efficient protein labelling inside the bacterial cytoplasm without apparent toxicity. The tris(triazolylmethyl)amine-based ligand BTTP significantly increased the redox potential of the coordinated Cu(I), sequestered Cu(I)-associated toxicity and dramatically accelerated the Cu(I)-catalysed 1,3-dipolar cycloaddition between azide- and alkyne-tagged molecules. By applying the power of this chemical transformation for compartment-specific protein labelling with a solvatochromic fluorophore, we developed a new technique for measuring acidity in different intracellular spaces of E. coli cells. When the extracellular pH dropped to 3, our cytoplasm- and periplasm-specific pH measurement showed an ~1.1 pH unit transmembrane pH gradient (ΔpH), which, in conjunction with the calculated membrane potential, allowed us to obtain the PMF value across the E. coli cytoplasmic membrane under this highly acidic condition. Our study revealed that E. coli cells actively maintain a pH gradient as well as a highly negative PMF value across its cytoplasmic membrane even under highly acidic conditions, which may be essential for acid-tolerance in Gram-negative bacteria. In addition, since PMF has important roles in energy production, cellular metabolism as well as bacterial motility, maintaining a relatively stable PMF in E. coli membrane under normal and stress conditions could be crucial in supporting diverse bacterial functions. We have recently extended the genetic code expansion strategy into a panel of pathogenic enteric bacteria species including Shigella and Salmonella [43] . These two pathogens developed effective but different acid-resistance systems to survive through the highly acidic mammalian stomach to cause infections in the small intestine. Transferring our pH indicator system into these pathogenic species for compartment-specific pH measurement under acid stress may shed light on their acid-resistance mechanisms. General materials Bacterial cells were grown in LB (Luria-Bertani) medium. Antibiotics were used at final concentrations of 50 μg ml −1 for ampicillin and 35 μg ml −1 for chloramphenicol (Sigma). E. coli bacteria strain DH10B was used for the expression of GFP and HdeA variant proteins. Chemical compounds BPS, TBTA, L -Histidine were purchased from Sigma-Aldrich, other compounds including ACPK, alk-4-DMN, BTTAA, BTTP and BTTPS were synthesized according to previous reports [11] , [12] , [24] , [25] . Expression of GFP protein containing ACPK in E. coli The plasmid pSupAR-Mb-ACPK-RS was co-transformed with a plasmid carrying the GFP-149TAG gene (pBAD-GFP-149TAG) into E. coli DH10B cells. Bacteria were grown at 37 °C in LB medium containing ampicillin (50 μg ml −1 ) and chloramphenicol (35 μg ml −1 ) for 3 h till OD 600 =0.6, at which point 1 mM ACPK (final concentration) was added to the culture. The bacteria were continuously grown at 37 °C for 30 min before being transferred to 30 °C for induction in the presence of 0.2% arabinose for 10 h. Cells were collected by centrifugation (10 min, 6,000 r.p.m., 4 °C). Proteins were extracted by sonication, and the extract was clarified by centrifugation (30 min, 13,000 r.p.m., 4 °C). The GFP protein containing ACPK was purified by HisTrap HP column (GE) operated with FPLC system (GE) according to standard protocols. In vitro labelling of GFP-ACPK mutant and SDS–PAGE analysis GFP protein containing ACPK was buffered to phosphate-buffered saline (PBS) buffer (pH 7.4) and diluted to a protein concentration of 30 μM. A total of 500 μl of GFP-ACPK in PBS buffer was reacted with alk-4-DMN (250 μM) at room temperature for 15 min in the presence of Cu(I)/ligand ([Cu]=50 μM, [ligand]=100 μM) and sodium ascorbate (2 mM). The reaction mixture was diluted to 5 ml with PBS and concentrated to 500 μl using an Amicon Ultra 3,000 MWCO centrifuge filter (Sigma), repeated four times to ensure that all the unreacted dye and Cu(I)/ligand were removed. The samples were analysed by SDS–PAGE: a 4–15% gel was run at 160 V and was imaged using ChemDoc for ultraviolet absorption before Coomassie blue staining. Biocompatible click-labelling inside bacterial cells E. coli cells expressing GFP (or HdeA) protein variants carrying the site-specifically incorporated ACPK handle were spun down and washed with PBS (pH 7.4) before being diluted into 0.5 ml PBS (OD 600 =0.6, containing 2% dimethyl sulphoxide). For the biocompatible CuAAC reaction, Cu(I)–ligand was added at a final concentration of 100 μM (100 μM CuSO 4 +200 μM ligands), while the sodium ascorbate was added at a final concentration of 2.5 mM. The final concentration of alk-4-DMN was 300 μM. The reaction was allowed to proceed at room temperature for 1 h with agitation and then quenched with bathocuproine disulphonate (5 mM). Cells were washed with PBS several times, and the samples were lysed for SDS–PAGE analysis or diluted in different buffers for flow cytometry analysis. In vitro detection of ROS production using coumarin-3-carboxylic acid A total of 5 mM coumarin-3-carboxylic acid was prepared as stock solution in DMF (N,N-dimethylformamide). CuSO 4 or CuSO 4 -ligands were prepared in PBS buffer at a concentration of 100 μM (200 μM ligands), then 2 mM sodium ascorbate was added. The mixture was incubated at room temperature for 15 min, then coumarin-3-carboxylic acid was added into the reaction buffer (100 μM). The samples were excited at 395 nm and the emission spectra were recorded from 400–600 nm. Cu(I)–BPS complex showed fluorescence upon 395-nm excitation, therefore it was not used in this assay. In vivo detection of ROS production using DCFH-DA The Cu(I)–ligands-treated (100 μM CuSO 4 +200 μM ligands, 2 mM sodium ascorbate, incubated at room temperature for 1 h) E. coli cells were collected and resuspended in PBS buffer (OD 600 =0.6), 5 μM (final concentration) of DCFH-DA (1 mM stock in dimethyl sulphoxide, Applygen Technologies Inc) were added to the cultures and incubated at room temperature in the dark for 30 min. DCFH-DA is a nonpolar dye which is converted into the polar derivative DCFH by cellular esterases. DCFH is nonfluorescent but switched to highly fluorescent DCF when oxidized by intracellular ROS or other peroxides, DCF has an excitation wavelength of 485 nm and an emission band between 500 and 600 nm. After incubation samples were transferred into a 96-well round-bottomed culture plate, and the fluorescence intensity was measured using a Synergy Hybrid plate reader (excitation: 485±15 nm, emission: 530±15 nm). Fluorescent measurements of Cu(I)–ligand-treated GFP GFP protein containing ACPK were buffered in PBS and diluted into a concentration of 30 μM (50 μl). Free Cu(I) or Cu(I)–ligand complex (50 μM CuSO 4 , 100 μM ligand) and 2 mM sodium ascorbate were added, and incubated at room temperature for 30 min. The Cu(I) was then removed by Micro Bio Spin-6 desalting column (Bio-Rad). The proteins were then diluted to 500 μl PBS buffer, transferred into a 96-well round-bottomed culture plate, and the fluorescence intensity was measured using a Synergy Hybrid plate reader (excitation: 480±15 nm, emission: 520±15 nm). PI staining assay of Cu(I)-treated E. coli cells The Cu(I)–ligands-treated (100 μM CuSO 4 +200 μM ligand, 2 mM sodium ascorbate, incubation at room temperature for 1 h) E. coli cells were collected and resuspended in PBS buffer (OD 600 =0.6), stained with PI (3 μg ml −1 ) and incubated at room temperature for 15 min. Cells were then washed with PBS three times, transferred into a 96-well round-bottomed culture plate and the fluorescence intensity was measured using a Synergy Hybrid plate reader (excitation: 535±20 nm, emission: 615±20 nm). Flow cytometry Analysis of cells by flow cytometry was carried out on a BD FACSCalibur Flow Cytometer equipped with a 488-nm laser. Fluorescence was detected in FL-1 channel for alk-4-DMN and FL-3 channel for trypan blue, fluorescence of DiOC 2 (3) was detected both in the FL-1 channel and FL-3 channel. After fluorescent labelling, the cells were washed with PBS four times and then diluted 1:1,000 in their respective buffers for fluorescence determination. Between 5 × 10 4 and 1 × 10 5 events were collected for each experiment; three parallel experiments were carried out for each sample. Data analysis was performed with CellQuest Pro software (BD Biosciences). Isolation of periplasmic and cytosolic proteins E. coli cells (in 10 ml culture) were collected by centrifugation at 6,000 r.p.m. for 5 min at 4 °C (ref. 44 ). The pellets were then resuspended in 0.5 ml buffer containing 10 mM Tris (pH 7.4), 1 mM EDTA, 15,000 U ml −1 Lysozyme, 20% (w/v) sucrose and incubated at room temperature for 10 min, 0.5 ml ice-cold water was then added and the sample was incubated on ice for an additional 5 min. Spheroplasts were collected by centrifugation (12,000 r.p.m., 5 min, 4 °C), and the supernatant was collected as the periplasmic fraction (peri-). The spheroplasts were resuspended in 0.5 ml buffer containing 10 mM Tris (pH 7.4), 1 mM EDTA and sonicated on ice for 5 min, and after centrifugation (12,000 r.p.m., 10 min, 4 °C), the supernatant was collected as the cytoplasmic fraction (cyto-). The samples were analysed by SDS–PAGE. Rabbit anti-HdeA (raised from rabbits) [45] and mouse anti-EF Tu (Santa Cruz Biotechnology) were used to verify this method. Electrochemical measurement Cu(I) complexes in ddH 2 O were made in situ by directly mixing the proper amounts (70 μl, 500 μM final concentration) of Cu(CH 3 CN) 4 PF 6 (I) solution (50 mM stock) in acetonitrile and the corresponding ligand in the cell (7 ml total volume) in a glove box under nitrogen [35] , [46] . Voltammetric measurements were carried out with CHI-660D electrochemical work station (ShangHai ChenHua). Experiments were performed at room temperature using a saturated calomel electrode as the reference electrode. The working electrode was a Pt electrode (ShangHai ChenHua, 3 mM diameter) and polished before experiment. Cyclic voltammetry was performed in the potential range of −0.6 to 0.6 V versus SCE at 50 mV s −1 . How to cite this article: Yang, M. et al . Biocompatible click chemistry enabled compartment-specific pH measurement inside E. coli . Nat. Commun. 5:4981 doi: 10.1038/ncomms5981 (2014).